A four-dimensional X-ray tomographic microscopy study of bubble growth in basaltic foam Understanding the influence of bubble foams on magma permeability and strength is critical to investigations of volcanic eruption mechanisms. Increasing foam porosity decreases strength, enhancing the probability of an eruption. However, higher porosities lead to larger permeabilities, which can lessen the eruption hazard. Here we measure bubble size and wall thickness distributions, as well as connectivity, and calculate permeabilities and tensile strengths of basaltic foams imaged by synchrotron X-ray tomographic microscopy during bubble growth in hydrated basaltic melts. Rapid vesiculation produces porous foams whose fragmentation thresholds are only 9–10 MPa and whose permeabilities increase from approximately 1×10 −10 to 1×10 −9 m 2 between 10 and 14 s despite decreasing connectivity between bubbles. These results indicate that basaltic magmas are most susceptible to failure immediately upon vesiculation and at later times, perhaps only 10's of seconds later, permeability increases may lessen the hazard of explosive, basaltic, Plinian eruptions. Rapid growth of bubbles in silicate magmas is the driving mechanism of volcanic eruptions [1] , [2] , but volcanic bubble growth cannot be directly observed, and instead vesicular ejecta provide samples of magmatic systems [3] . However, the exact timing of bubble formation and bubble growth rates may be obscured by syn- and post-eruption processes [3] , [4] . To circumvent these limitations, bubble growth in the laboratory was studied by quenching techniques [5] , [6] , [7] , by analogue studies [8] and by in situ studies during 1 atm degassing (for example, see ref. 9 ). Unfortunately, these studies investigated bubble growth at relatively long durations, 10 2 –10 5 s, whereas the first seconds of bubble growth critically influence volcanic eruption mechanisms. We investigated the first 10–18 s of bubble growth in a basaltic system using a laser-based heating system [10] along with an ultrafast endstation at the TOMCAT tomographic microscopy beamline of the Swiss Light Source (Villigen, Switzerland) to obtain four-dimensional, ( x , y , z and time) microstructural information. We measured the evolution of bubble size distributions and the corresponding distributions of wall numbers and thickness between the bubbles that hold the magma together. We also modelled changes in permeability with bubble growth through lattice-Boltzmann simulations and variations in relative tensile strength by application of a fibre bundle model [11] . We chose a basaltic composition with either 3 or 7 wt.% dissolved H 2 O to study because although basaltic volcanism is dominated by effusive, low-intensity eruptions, some basaltic volcanoes can violently erupt in explosive, Plinian events [12] , [13] and the mechanisms by which a basaltic volcano switches from non-violent to violent eruptions remain enigmatic. General observations Hydrated glasses were heated on the TOMCAT beamline to above their glass transition, ~600 °C, in <30 s using the laser furnace. Then, as temperatures increased to ~1,200 °C, full three-dimensional (3D) data sets were collected every second for 18 s (as described in the Methods section). The rapidity of the heating simulates instantaneous decompression, which is estimated using a water solubility model [14] to be ~90 MPa for the water-poor experiment with 3 wt.% H 2 O and 450 MPa for the water-rich one with 7 wt.% H 2 O. We report measurements commencing 10–11 s following the start of bubble growth because the dynamics of earliest bubble growth result in rapid sample movement, occurring faster than the temporal resolution of the scan (as seen in the image slices displayed in Supplementary Figs S1 and S2 ). Experiments are limited to a maximum duration of 18 s because of data acquisition limitations of the system combined with observations of sample deflation during later stages of the experiments. This experimental duration is similar to the estimated 10-s growth duration of bubbles in Hawaiian eruptions [15] . Interior 1.19×1.19×0.89 mm 3 volumes (400×400×300 voxels; Fig. 1 ) were used for analysis because of differences observed between the centres and the edges of the samples that are attributed to enhanced volatile loss at the surface ( Fig. 1 ; Supplementary Figs S1 and S2 ; Supplementary Movies 1 and 2 ). Samples were analysed [16] and bubble numbers and volumes, as well as pore throat sizes and wall thicknesses, were measured based on 3D skeletonization ( Fig. 2 ; Methods). 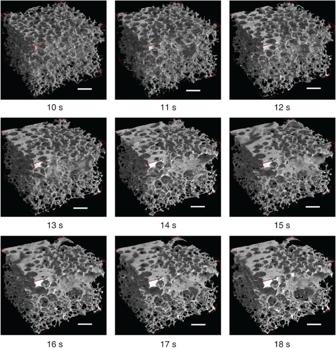Figure 1: Bubble growth in a basaltic melt at 1 atm. Volume renderings showing bubble growth in the central portion (1.19×1.19×0.89 mm3, 400×400×300 voxels) of the water-poor (3 wt.%) sample co-010b from 10 to 18 s after the start of bubble growth. The scale bar in each image corresponds to ~200 ìμm and changes from front to back and top to bottom of the sample because of the perspective view in each image. Figure 1: Bubble growth in a basaltic melt at 1 atm. Volume renderings showing bubble growth in the central portion (1.19×1.19×0.89 mm 3 , 400×400×300 voxels) of the water-poor (3 wt.%) sample co-010b from 10 to 18 s after the start of bubble growth. The scale bar in each image corresponds to ~200 ìμm and changes from front to back and top to bottom of the sample because of the perspective view in each image. 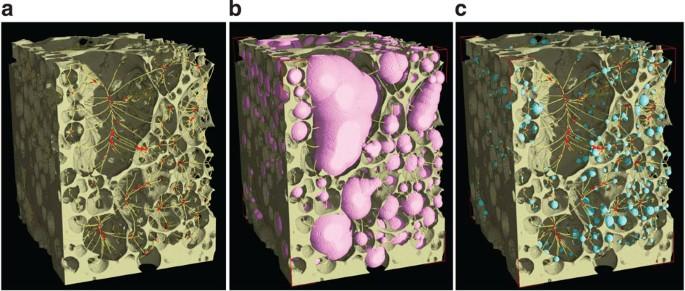Figure 2: Example of skeletonization techniques used to measure bubble and pore throat sizes. (a) The topology preserving skeleton with nodes shown in red at the intersections of the branches. (b) The maximal inscribed spheres used to calculate the bubble volumes. (c) The maximal inscribed spheres used to calculate the pore throat diameters. Wall thicknesses were also determined using maximal inscribed spheres. Full size image Figure 2: Example of skeletonization techniques used to measure bubble and pore throat sizes. ( a ) The topology preserving skeleton with nodes shown in red at the intersections of the branches. ( b ) The maximal inscribed spheres used to calculate the bubble volumes. ( c ) The maximal inscribed spheres used to calculate the pore throat diameters. Wall thicknesses were also determined using maximal inscribed spheres. Full size image Bubble number densities (BNDs) The BND decreases from a few hundred down to ~100 mm −3 between 10 and 14 s in both samples, then becomes approximately constant for the water-rich sample and slowly drops for the water-poor sample ( Fig. 3a,b ; Table 1 ). The 10–14 s data demonstrate an exponential decrease of the BND with time that when extrapolated back to zero-time yield an initial BND of ~19,000 mm −3 for the water-rich sample and ~6,200 mm −3 for the water-poor one ( Supplementary Fig. S3 ), consistent with the greater supersaturation of the water-rich sample during initial bubble growth at 1 atm [17] . The decrease in the BND results from coalescence of many small bubbles to form a few larger ones with volumes between ~10 6 and 10 8 μm 3 , as can be observed in the tomographic images ( Figs 1 and 3a,b ). The BNDs of ~100 mm −3 are similar to measurements of scoria from Hawaiian fire fountains [15] , Villarica scoria and pumice [18] , and normal Strombolian eruptions [4] , whose BNDs vary from 60 to 200 mm −3 . The initial BNDs are similar to those seen in products of basaltic, Plinian and sub-Plinian eruptions [4] , [12] , [13] , [19] , ~10,000 mm −3 . 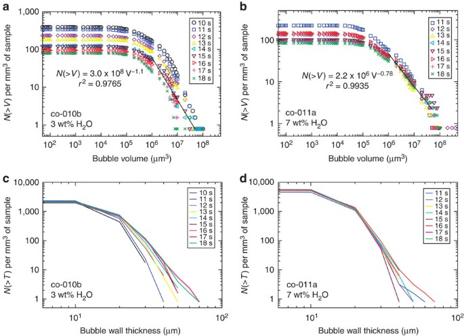Figure 3: Cumulative bubble size and bubble wall thickness distributions during bubble growth. (a) Cumulative bubble size distributions for the water-poor (3 wt.%) sample from 10 to 18 s of growth. (b) Cumulative bubble size distributions for the water-rich (7 wt.%) sample from 11 to 18 s of growth. Inaandb,Nis the number of bubbles andVis the bubble volume;r2is the correlation coefficient of the power law fit to the bubble size distributions at 14 s of growth. (c) Cumulative wall thickness distributions for the water-poor sample from 10 to 18 s of growth. (d) Cumulative wall thickness distributions for the water-rich sample from 11 to 18 s of growth. Incandd,Nis the number of bubble walls andTis the bubble wall thickness. Figure 3: Cumulative bubble size and bubble wall thickness distributions during bubble growth. ( a ) Cumulative bubble size distributions for the water-poor (3 wt.%) sample from 10 to 18 s of growth. ( b ) Cumulative bubble size distributions for the water-rich (7 wt.%) sample from 11 to 18 s of growth. In a and b , N is the number of bubbles and V is the bubble volume; r 2 is the correlation coefficient of the power law fit to the bubble size distributions at 14 s of growth. ( c ) Cumulative wall thickness distributions for the water-poor sample from 10 to 18 s of growth. ( d ) Cumulative wall thickness distributions for the water-rich sample from 11 to 18 s of growth. In c and d , N is the number of bubble walls and T is the bubble wall thickness. Full size image Table 1 Summary of measurements and simulation results. Full size table Vesicularities The measured vesicularity of the water-poor sample is between 0.86 and 0.87 and that of the water-rich sample between 0.79 and 0.81 ( Table 1 ). The vesicularity difference between the samples is attributed to stochastic processes (for example, more rapid formation of a percolating cluster) that resulted in greater water loss from the water-rich sample before maximum bubble growth could occur. The experimental vesicularity is similar to natural basaltic scoria (70–95%) produced in eruptions with mass eruption rates of 10 3 –10 8 kg s −1 (ref. 19 ). Radial growth rates of approximately 1–10 μm s −1 were estimated (see Methods ), similar to the estimated growth rate of 9 μm s −1 for bubbles in Hawaiian fire fountains [15] . The maximum vertical expansion rate measured was 2×10 −4 m s −1 and the corresponding strain rate was 0.1 s −1 (see Methods ). Bubble size distributions Although the bubble size distribution at each different time step can be fit by slightly different power laws, all can be described by a power law with an exponent of ~1 for bubble volumes between 10 6 and 5×10 7 μm 3 ( Fig. 3a,b ). In detail, the exponents of the water-poor sample vary from 1.1 to 1.5 and for the water-rich sample from 0.6 to 1. The stationary location of the break in the horizontal portion of the distributions with time ( Fig. 3a,b ) is evidence against the presence of Ostwald ripening [15] in these experiments. Furthermore, the rapid drop in the BND seen in Fig. 3 is also inconsistent with Ostwald ripening [7] . Both experiments' power-law bubble size distributions are indicative of far-from-equilibrium behaviour [7] , [9] , [20] , [21] . However, the water-poor experiments showed slightly higher power-law exponents and greater deviations from power-law behaviour at longer growth durations ( Fig. 3a,b ), suggestive of its entrance into the decaying coalescence regime [20] and evolution towards equilibrium exponential distributions [7] , [9] . The experimental power-law exponents are similar to those of natural scoria from normal Strombolian eruptions in the same volume range [4] , ~1. These exponents are only a little below those of the same size range of vesicles in Stromboli sub-Plinian pumice [4] , of scoria from the basaltic, Fontana Plinian eruption [12] and from the 122 BC basaltic, Plinian eruption of Etna [13] , which when expressed as volume are each ~1.5. Bubble wall thickness and connectivity The number of bubble walls per mm 3 for the water-poor experiment is ~2,000, and walls with a thickness of 20 μm and greater increase significantly with time ( Fig. 3c ). In contrast, the water-rich experiment has ~5,000 walls per mm 3 , and the number of thicker walls demonstrates only a small increase with time ( Fig. 3d ). The maximum bubble wall thickness in both samples varies between 30 and 70 μm. The pore throat diameters linking bubbles vary from approximately 6 to 100 μm and their distributions are exponential, with the exception of the first ones in the water-rich sample time series, which display power-law behaviour ( Supplementary Fig. S4 ). The connective density, β , in both samples decreases with time, from 4.4 to 1.9×10 6 mm −3 for the water-poor experiment and from 7.5 to 2.4×10 5 mm −3 in the water-rich one (Methods; Table 1 ). The decreases in β can be qualitatively observed in Fig. 1 , where walls between bubbles become more evident with increasing duration. Changes in β are most pronounced at growth durations less than 14 s. The decrease in β for the water-poor sample is correlated with a decrease in the average coordination number from 8.3 to 5.1 ( Table 1 ). However, the average coordination number for the water-rich sample remains approximately constant, only varying from 4.1 at 11 s to 3.9 at 18 s. Permeabilities Despite the nearly constant porosity during growth, the textural evolution of these samples affect Darcian permeabilities, which were calculated at 10 s (water-poor) or 11 s (water-rich), 14 and 18 s using lattice-Boltzmann simulations (see Methods ). During bubble growth the permeability of each sample increases by an order of magnitude from 1.5×10 −10 to 1×10 −9 m 2 , with most of the change occurring between the first two time steps modelled, where the permeability of the water-poor sample increases from 1.5×10 −10 m 2 at 10 s to 5.3×10 −10 m 2 at 14 s, and the permeability of the water-rich sample increases from 2.1×10 −10 m 2 at 11 s to 8.6×10 −10 m 2 at 14 s ( Table 1 ). The permeability trend indicates that the growth of larger vesicles, between 10 6 and 10 8 μm 3 , which enhance permeability [22] , overwhelms the approximately 2.5 x drop in β . This interplay between the bubble size distribution and the connective density indicates that measurement of vesicularity alone is not enough to predict permeability and may explain some of the observed differences in porosity–permeability relationships reported in the literature [21] . Failure modelling The fibre bundle model (see Methods ) was used to characterize the strength of foam and the manner in which it fails. The quantities of interest are the force per fibre, σcrit and the proportion of remaining fibres to the initial fibres, U , at critical failure of the bundle. The time-averaged σcrit (average with 2 s.d.) for the water-poor sample is 1.83±0.01×10 −4 and is 1.61±0.01×10 −4 for the water-rich one. The increase in the number of thicker bubble walls with growth duration ( Fig. 3c,d ) might be expected to increase the strength of the samples, but both samples only displayed small variations in σcrit with time, as reflected by the small standard deviations about the mean. Converting these strengths to differential pressures at failure (see Methods ) yields fragmentation threshold pressures of 10.5 MPa for the water-poor sample and 9.2 MPa for the water-rich one, consistent with experimental measurements [23] , [24] . The average values of U for the samples are almost indistinguishable, for the water-poor sample it is 0.739±0.018 and for the water-rich one it is 0.741±0.037. Importantly, the model demonstrates that failure occurs after only ~25% of the fibres fail, and these are the weakest ones in each bundle. The similar vesicularities, BNDs, growth rates, size ranges and power-law distributions of these experiments and those of natural samples [4] , [12] , [13] , [15] , [18] , [19] suggest that even though the temperature–pressure path of the experiments did not exactly mimic nature, they provide insight into magmatic processes. These experiments demonstrate that bubble growth in basaltic melts occurs virtually instantaneously when the samples are supersaturated and above the glass transition. Thus, no delay in bubble growth is expected in basaltic systems and they should vesiculate rapidly when supersaturated with as little as 3 wt.% water; there is no support for the suggestion that delayed bubble nucleation has a role in basaltic Plinian eruptions [12] . The vesiculation of supersaturated basaltic melts to porosities greater than 0.8 in less than 11 s in these experiments also is evidence against the existence of a fixed fragmentation threshold of approximately 0.75–0.80 vesicularity [25] . The measured radial growth rates of approximately 1–10 μm s −1 and strain rate of 0.1 s −1 are orders of magnitude too slow to cross the glass transition and cause fragmentation [26] . And, the rates of bubble growth and expansion, 2×10 −4 m s −1 , are not rapid enough to cross the inertia-driven fragmentation threshold proposed for low-viscosity basaltic melts [27] . The experiments indicate that initial BNDs are similar to those seen for basaltic, Plinian eruptions and suggest the possibility that all vesiculating basaltic magmas with moderate water concentrations can potentially form Plinian eruptions because of the observed correlations between BND and explosivity [4] , [19] . However, most basaltic eruptions are known for their relatively quiescent behaviour and effusive eruptions are most common, although Strombolian eruptions and Hawaiian-type fire fountaining are not rare [3] . Thus, the experiments behave similarly to most basaltic eruptions; they display slow growth of bubbles without a suggestion of explosive behaviour. But, the question remains: How did the experiments (and potentially most natural magmas) evade a state (the proto-Plinian state) where they could fail and form Plinian eruptions? These experiments and simulations demonstrate that in this case any proto-Plinian state must occur within the first 10 s of bubble growth and during a time when porosity is rapidly increasing and sample strength is rapidly falling. The lack of failure in these experiments requires that the permeability increases faster than the strength decreases, as a difference of only 9–10 MPa in pressure between the bubbles and their surrounding environment is enough for catastrophic failure of these experiments after 10 s of bubble growth. Although we could not determine permeability at the earliest times of these experiments, previous work indicates that Stromboli magmas reach permeabilities sufficiently high to lose their gas at porosities near 0.3 (ref. 21 ), or less than one-half of the porosities measured after 10 s, and magmas with 0.3 porosity display fragmentation thresholds similar to those calculated at high porosities [23] , [24] . What appears to be required to form Plinian eruptions is a mechanism by which the permeability can be maintained at low values, probably orders of magnitude below the minimums found here of ~10 −10 m 2 , for only a short time as the magma weakens. The presence of crystals has been suggested as the mechanism to prevent the increase of permeability as strength decreases [12] , [13] , but measurements of crystal- and bubble-bearing vesiculated Stromboli magmas indicate that crystals increase permeabilities at vesicularities of 0.3–0.5 and have no measurable effect at high vesicularities [28] . Although we are hesitant to eliminate totally the role crystals may have in Plinian eruptions, particularly at low porosities, the available evidence points towards the importance of bubble growth rate, which strongly influences magma ascent rates and therefore decompression rates, as the controlling variable that determines whether a basalt magma erupts effusively, or in a Plinian manner. The required exit velocities for the inertial fragmentation [27] of low-viscosity basaltic magmas are approximately 10 −2 –10 −1 m s −1 . The growth velocities of the experiments were 10 −4 m s −1 ; therefore the lack of failure in the experiments is consistent with, and provides support for, the inertial fragmentation hypothesis. In conclusion, these experiments suggest that catastrophic failure of a basaltic, magmatic foam and formation of a Plinian eruption are most likely to occur immediately on vesiculation and rapid decompression and be caused by rapid bubble expansion leading to inertial fragmentation. But, if the magma survives without erupting for perhaps as little as 10 s after vesiculation, the permeability may increase sufficiently to allow magma degassing and lower the threat of failure and eruption. This latter case appears to be the norm for basaltic eruptions and explains why effusive eruptions of basalts are common and Plinian ones are rare. Sample preparation Powder of high-potassium basalt from the 2003 paroxysmal eruption of Stromboli volcano (Italy) was used to synthesize starting glasses (composition in ref. 21 ). Approximately 70 mg of powder plus distilled water (3 wt.% H 2 O for water-poor co-010b and 7 wt.% for water-rich co-011a) were loaded into 3 mm diameter Pt tubes and welded closed. The mixtures were melted in a piston-cylinder apparatus at 1,250 °C, 1.0 GPa for 1 h in 19.1 mm NaCl-pyrex assemblies [29] and quenched isobarically to produce hydrated, crystal-free glasses. In situ X-ray tomographic microscopy X-ray tomographic microscopy was performed at the TOMCAT beamline of the Swiss Light Source at the Paul Scherrer Institute (Villigen, Switzerland) using a laser-based heating system [10] and an ultrafast endstation [30] . Two class-four diode lasers (980 nm) were placed 180° apart and ~40 mm from the sample. The lasers are each capable of providing 150 W of power; a pyrometer measured sample temperature. Lasers were pointed just below the sample holder on the zirconia rod that connected the sample holder to the rotation stage until the sample reached ~600 °C, at which point the hydrated glass sample was lowered into the laser beam and rapidly heated to between ~1,150 and 1,200 °C during data acquisition. Polychromatic X-rays were filtered to 5% transmission, generating 1 ms exposure times, and 951 projections were captured over 180° of rotation. The ultrafast endstation incorporates a PCO.Dimax camera, which acquires and transfers data orders of magnitude faster than CCD cameras. The detector used for these scans incorporated an optical microscope, designed specifically for high numerical apertures and polychromatic radiation, with an adjustable magnification tuned to fourfold for this experiment. This corresponds to a pixel size of 2.98×2.98 μm 2 and a field of view of 6.0×6.0 mm 2 . The optics were coupled to LuAG:Ce 100 μm thick scintillator screen. Reconstructions were performed by using the GRIDREC algorithm [31] , [32] coupled with parzen filtering of the sinograms. Image analysis and quantification Data collected at TOMCAT were quantitatively analysed with the Pore3D software library [16] . An edge preserving smoothing filter was applied, followed by a fixed-threshold to separate pore space (bubbles) from glass. Descriptors based on skeleton analysis [33] were used to derive pore- and throat-size distributions and wall thickness measurements. The skeleton of any 3D object is intuitively the 'spine' of the object running along its geometric middle, which consists of a graph of nodes and branches ( Fig. 2 ). The skeletonization algorithm of Brun and Dreossi [34] was adopted; pore and throat thickness measures were computed using the concept of maximal inscribed sphere [35] . Skeleton nodes correspond to pore bodies and branches of the skeleton correspond to the channels connecting the pores. A pore/node correction was applied as several skeleton nodes may occur in the same pore body [36] . The coordination number is the average of the number of branches per node in the skeleton. Radial growth rates were calculated from the radii of the larger bubbles divided by experimental duration. The average connectivity, or connective density, β , is calculated from the number of skeleton nodes (bubbles) and branches (pore throats): β =[1−(nodes−branches)]/sample volume. Bubble wall thickness was measured as the average diameter of septa separating two bubbles using a maximal inscribed sphere construction [37] . Bubble, pore throats and wall thickness measurements were plotted as cumulative distributions because of the discontinuous nature of the measured data resulting in many size categories (or bins) containing no objects [20] , [38] in order to determine their type of distribution (exponential versus power law). Cumulative distributions are preferable to probability distributions because the former are a stable series of a progressively increasing sum, or decreasing difference, from which the probability distribution function can be easily calculated [39] . The vertical expansion rate of the sample was determined by measuring the heights of the central portion of each experimental sample at each of the 18-time steps from the start until the end of the experiment and from these heights the rate was calculated. However, because of image blurring at earlier times during growth these measurements are only considered accurate to within a factor of 3. These measurements were then used to calculate the strain rate with respect to the original sample. Lattice-Boltzmann modelling of permeabilities Because of the dynamic nature of the experiments and the collapse of the samples and loss of vesicularity near their termination, sample permeabilities could not be measured. Instead, lattice-Boltzmann modelling of permeabilities was performed using a modified version of an established code [40] , [41] . Details of the permeability modelling can be found in ref. 21 , in which the accuracy of the Darcian permeabilities calculated by modelling was directly compared against measured permeabilities. Because of computer limitations, central subvolumes of 200×200×200 voxels were chosen from the 400×400×300 volumes for modelling. Permeabilities of the water-poor sample at 10, 14 and 18 s duration in the x -, y - and z -directions were calculated. Because no significant permeability differences between the directions were noted at any individual time step, all of the values at each time step were averaged ( Table 1 ). The same procedure was followed for the water-rich sample, except that permeabilities at 11, 14 and 18 s were calculated and averaged ( Table 1 ). Fibre bundle tensile strength modelling The relative tensile strength of the samples at each time step was modelled with the Global Load Sharing (GLS) fibre bundle model [11] . This model was chosen because both the fibre bundle model and magmatic foam failure are caused by tensional forces and the walls between the expanding bubbles can be considered analogous to the fibres in the modelled bundle. This numerical model does not yield absolute strengths, but provides relative strength measures of a sample as it changes. The conceptual model consists of a bundle of fibres, described by their squared widths (which correlate linearly with tensile strength), attached to two parallel plates. A force, F , is applied to separate the plates and under GLS this force is distributed evenly among all fibres in the bundle; the force per fibre, σ , equals F / N , where N is the total number of fibres. All fibres with squared widths, or tensile strengths, less than σ break. The force per remaining fibre is then recalculated as σ = F / N rem , where N rem is the number of remaining fibres after the failure event, and the process iterated until either failure ceases or the bundle catastrophically fails. This model was implemented using a code in the C-language and verified to ensure that it reproduced previous results [11] . The relative strengths calculated by the model were converted to the fragmentation thresholds of vesicular rocks. Experiments [23] define a relationship between the fragmentation threshold, expressed as the pressure difference between the inside and outside of a sample at fragmentation, Δ P (in MPa), and the porosity: Δ P =75.367 φ −0.76446 , where φ is expressed in percent. The average relative tensile strength calculated of a reference sample with only 2.5% porosity (co-005a) was equated with the Δ P -value calculated from the relationship between Δ P and φ , yielding a relationship between the tensile strengths calculated by the fibre bundle model and experimentally determined Δ P -values. With this relationship, the fragmentation thresholds of the two samples in this study could then be calculated from their relative tensile strengths using co-005a as a reference. How to cite this article: Baker, D.R. et al . A four-dimensional X-ray tomographic microscopy study of bubble growth in basaltic foam. Nat. Commun. 3:1135 doi: 10.1038/ncomms2134 (2012).